Osteoblast-derived vesicles induce a switch from bone-formation to bone-resorption in vivo Bone metabolism is regulated by the cooperative activity between bone-forming osteoblasts and bone-resorbing osteoclasts. However, the mechanisms mediating the switch between the osteoblastic and osteoclastic phases have not been fully elucidated. Here, we identify a specific subset of mature osteoblast-derived extracellular vesicles that inhibit bone formation and enhance osteoclastogenesis. Intravital imaging reveals that mature osteoblasts secrete and capture extracellular vesicles, referred to as small osteoblast vesicles (SOVs). Co-culture experiments demonstrate that SOVs suppress osteoblast differentiation and enhance the expression of receptor activator of NF-κB ligand, thereby inducing osteoclast differentiation. We also elucidate that the SOV-enriched microRNA miR-143 inhibits Runt-related transcription factor 2, a master regulator of osteoblastogenesis, by targeting the mRNA expression of its dimerization partner, core-binding factor β. In summary, we identify SOVs as a mode of cell-to-cell communication, controlling the dynamic transition from bone-forming to bone-resorbing phases in vivo. Bone remodeling occurs in different parts of the body throughout life to maintain bone architecture balance and systemic mineral homeostasis. During this “remodeling” process, osteoclasts remove mineralized bones, whereas osteoblasts form new bones [1] , [2] , [3] . These resorption and formation phases are linked and balanced with intermittent coupling phases. Functional coupling between these two cell types is critical for the maintenance of proper bone metabolism, and the mechanisms controlling the transition from bone-resorbing to bone-forming phases (i.e., reversal phase) have been investigated [4] , [5] , [6] . These mechanisms are regulated by insulin-like growth factor I and transforming growth factor-β released from the bone matrix during bone resorption [5] , sphingosine-1-phosphate [7] , collagen triple helix repeat containing 1 [8] , Semaphorin 4d [9] , ephrin B2 [10] , and receptor activator of NF-κB ligand (RANKL)/RANK reverse signaling [11] . Notably, all of these factors contribute to the transition from bone-resorbing to bone-forming phases. Nevertheless, the molecular and cellular mechanisms terminating osteoblastic bone formation and promoting osteoclastic bone resorption (i.e., “reciprocal” reversal phase) remain elusive. Intravital optical imaging using multiphoton microscopy can help dissect in vivo cellular dynamics in various intact tissues and organs [12] , [13] , [14] . To understand the spatiotemporal dynamics of bone remodeling in vivo, we established an intravital imaging technique to visualize the intact bone tissues of living mice [15] , [16] , [17] , [18] . Using this method, we explored the interplay between bone-destroying osteoclasts and bone-forming osteoblasts and found that direct cell-to-cell contact led to the inhibition of osteoclastic bone resorption [19] . However, the spatial resolution of intravital bone imaging was insufficient to visualize structures smaller than cells. In this study, we established an advanced high-resolution microscopy system to visualize extracellular vesicles secreted and captured by mature osteoblasts (mOBs) in vivo. We identified a subset of mOB-derived vesicles limiting bone formation and stimulating osteoclastogenesis, thus regulating the “reciprocal reversal phase,” through a microRNA (miRNA)-mediated mechanism. Visualization of small osteoblast-derived vesicles We have previously generated reporter mice expressing enhanced cyan fluorescent protein (ECFP) in mOBs driven by a 2.3 kb fragment of rat type I collagen α promoter (Col1a1*2.3) (Col2.3-ECFP mice). In this reporter line, ECFP is expressed in bone-forming mOBs but not in immature osteoblasts [19] . We performed intravital multiphoton imaging using high spatial resolution to visualize bone tissues in Col2.3-ECFP mice, and observed many ECFP-positive vesicles in the vicinity of the cell bodies of mOBs (Fig. 1a–c ). Tracking analyses showed that the small osteoblast vesicles (SOVs) had a diameter of ≤1 µm and had a higher speed than large osteoblast vesicles (LOVs), which were >1 µm in diameter (Fig. 1d ). Moreover, time-lapse imaging revealed that SOVs were released to the extracellular space and were taken up by mOBs in vivo within ~20 min (Fig. 1e, f ; Supplementary Video 1 ). SOV release and uptake were also observed in vitro in primary osteoblasts from Col2.3-ECFP mice (Fig. 1g–j ; Supplementary Videos 2 , 3 ). The uptake of SOVs by mOBs was confirmed by co-culture of mOBs and membrane-labeled SOVs (Supplementary Fig. S1a–c ; Supplementary Videos 4 , 5 ). We also found that SOVs expressed CD63, a marker of extracellular vesicles [20] (Supplementary Fig. S1d, e ). These results suggest that mOBs actively secrete and take up SOVs both in vivo and in vitro, communicating via extracellular SOVs in a paracrine or autocrine manner. Fig. 1: Communication among osteoblasts via small osteoblast vesicles in vivo and in vitro. a Schematic representation of mouse skull bone (left) and an intravital multiphoton, maximum-intensity projection image of skull bone tissues from Col2.3-ECFP mice (a representative image, at least three independent experiments) (right). Cyan: mature osteoblasts (mOBs) and extracellular vesicles (EVs) from mOBs; blue: bone surface, second harmonic generation. Scale bar: 20 μm. b Three-dimensional image of visual field shown in ( a ). Arrowhead indicates an EV. Scale bar: 20 μm. c Magnified view of region outlined in ( a ). Arrowheads indicate EVs. Scale bar: 10 μm. d Speed of mOB-derived EVs by tracking analysis of EVs shown in ( c ) ( n = 51). SOVs: small osteoblast vesicles with a diameter of ≤1 µm; LOVs: large osteoblast vesicles with a diameter of >1 µm. e Consecutive time-lapse images of SOVs released by mOBs indicated by yellow lines in ( c ). Arrowheads and dotted lines indicate SOVs and their tracks, respectively. Scale bar: 5 µm. f Consecutive time-lapse images of SOVs taken up by mOBs indicated by dotted lines in ( c ). Arrowheads and dotted lines indicate SOVs and their tracks, respectively. Scale bar: 5 µm. g , h Representative images of primary osteoblasts of Col2.3-ECFP mice of at least three independent experiments. Cyan: mOBs and mOB-derived EVs. Scale bar: 20 µm. i Consecutive time-lapse images of released SOVs indicated by yellow lines in ( g ). Arrowheads and dotted lines indicate SOVs and their tracks, respectively. Scale bar: 10 µm. j Consecutive time-lapse images of internalized SOVs indicated by dotted lines in ( h ). Arrowheads and dotted lines indicate SOVs and their tracks, respectively. Scale bar: 10 µm. Full size image SOVs of approximately 400 nm in diameter suppress osteoblast differentiation To characterize SOVs, we performed electron microscopy and nanoparticle tracking analyses to evaluate the morphology and size distribution of isolated SOVs from primary osteoblasts (Fig. 2a–e ). Electron microscopy showed that the diameter of SOVs ranged from 100 nm to 1 µm, and that the structures and electron densities of SOVs varied (Fig. 2b ). Nanoparticle tracking analyses revealed two peaks associated with different SOV sizes: one around 200 nm in diameter (hereafter called SOV-F1) and one around 400 nm in diameter (hereafter called SOV-F2) (Fig. 2c ). SOV-F1 were isolated by 0.22-µm filtration (Fig. 2a ); the collected SOV-F1 had similar sizes and electron densities (Fig. 2d, e ). As the SOVs observed by intravital imaging ranged in size from 0.26 to 1 µm, they were likely SOV-F2. Fig. 2: SOV-F2 inhibits osteoblast differentiation. a Schematic representation of SOV isolation via differential centrifugation. F1: fraction 1; F2: fraction 2. b Transmission electron micrograph of total SOVs (at least three independent fields from 1 mouse). Scale bar: 1 µm. c Nanoparticle tracking analysis of total SOVs (at least three independent experiments). d Transmission electron micrograph of SOV-F1 after 0.22 µm filtration (at least three independent fields from 1 mouse). Scale bar: 500 nm. e Nanoparticle tracking analysis of SOV-F1 after 0.22 µm filtration (at least three independent experiments). f Runx2 , Sp7 , Col1a1 , and Bglap mRNA levels in osteoblasts treated with PBS, total SOVs (F1 + F2), or SOV-F1 ( Runx2 , Sp7 and Bglap : n = 5; Col1a1 : n = 6 biological replicates per group). g , h ALP activity in osteoblasts treated with PBS, total SOVs (F1 + F2), or SOV-F1 ( n = 6 biological replicates per group). Representative images ( g ) and quantitative analysis ( h ) Scale bar: 10 mm. i Percentages of 7-AAD-positive apoptotic cells among CD45-negative primary osteoblasts at 6 days after treatment with PBS, total SOVs (F1 + F2), or SOV-F1 ( n = 3 biological replicates per group). Data are means ± SEMs. Statistical significance was determined by one-way ANOVA with Dunnett’s multiple comparison post hoc test ( f , h , i ). Full size image Extracellular vesicles are composed of a lipid bilayer containing transmembrane proteins, as well as enclosed cytosolic proteins and RNAs (especially mRNAs and miRNAs). Extracellular vesicles are thought to serve as a mode of communication among neighboring or distant cells [21] , [22] . Here, we investigated the role of SOVs in the communication of neighboring osteoblasts. The relative expression levels of genes related to osteoblast differentiation in primary osteoblasts were analyzed 2 days after treatment with phosphate-buffered saline (PBS), total SOVs (F1 + F2), or SOV-F1 (Fig. 2f ). The expression levels of runt-related transcription factor 2 ( Runx2) and Osterix (also known as Sp7 ), master transcription factors involved in osteoblast differentiation [23] , [24] , [25] , as well as those of the osteoblastic matrix proteins type 1 collagen ( Col1a1 ) and osteocalcin (also known as Bglap ), were significantly lower in the SOV-treated group than in the PBS control group (Fig. 2f ). Total SOVs (F1 + F2) were more potent than SOV-F1 in suppressing the expression of osteoblast-related genes, suggesting that large SOVs mediate this transcriptional regulation. Consistently, in the osteoblastic cell line MC3T3-E1, the relative mRNA levels of Runx2 and Sp7 were significantly lower in the total SOV-treated group than in the PBS control group in a dose-dependent manner (Supplementary Fig. S2a ). SOV-F1 treatment moderately affected the expression of Runx2 but not the expression of Sp7 (Supplementary Fig. S2b ). To exclude the effects of proteins and RNAs outside the extracellular vesicles, such as membrane fragments and anchor proteins on the SOV membrane, we examined whether proteinase K and/or RNase treatment modulated the effects of SOVs on Runx2 and Sp7 expression. Inhibition by SOVs was unaffected by RNase and proteinase K (Supplementary Fig. S2c ) [26] , indicating that components in SOVs, but not protein and RNA contaminants outside SOVs, were responsible for the inhibition of Runx2 and Sp7 expression. We performed alkaline phosphatase (ALP; Alpl ) staining to assess bone-forming activity in SOV-treated cells. ALP activity was significantly suppressed in the total SOV-treated group but not in the SOV-F1-treated group (Fig. 2g, h ). We also assessed collagen production and mineralization by SOV-treated osteoblasts by Fast Green/Sirius Red staining and Alizarin Red S staining, respectively. Collagen production and mineralization by total SOV-treated osteoblasts were inhibited, compared with PBS control and SOV-F1-treated osteoblasts (Supplementary Fig. S2d, e ). Next, we analyzed the effect of SOVs on cell death using 7-amino actinomycin D (7-AAD) staining; however, we found no significant differences among the groups (Fig. 2i ). These results suggest that total SOVs (F1 + F2), but not SOV-F1, suppress osteoblast differentiation without affecting cell viability. SOV-treated osteoblasts promote osteoclastogenesis Osteoblast-lineage cells produce RANKL, encoded by the Tnfsf11 (also known as Rankl ) gene, an essential factor for osteoclastogenesis [27] , [28] , and osteoprotegerin ( Opg ), a decoy receptor for RANKL [28] , [29] , to regulate osteoclast differentiation and function. Therefore, we investigated the roles of SOVs in the expression of Rankl and Opg . The expression level of Rankl was significantly higher in the total SOV-treated group than in the PBS control group. In addition, the expression level of Opg was significantly lower in the total SOV-treated group than in the PBS control group. However, SOV-F1 did not affect Rankl or Opg expression (Fig. 3a ). These results suggested an increased osteoclastogenic potential in total SOV-treated mOBs. Therefore, we assessed osteoclast differentiation using bone marrow macrophages (BMMs) co-cultured with either total SOV-treated osteoblasts or PBS-treated osteoblasts. When starting the co-culture, we washed out SOVs with culture medium to prevent SOVs from directly affecting BMMs. Tartrate-resistant acid phosphatase (TRAP)-positive mature osteoclasts (mOCs) were generated within 3 days of co-culture of BMMs with total SOV-treated osteoblasts without additional supplementation of recombinant RANKL. In contrast, no significant mOC generation was observed when BMMs were co-cultured with PBS-treated osteoblasts (Fig. 3b, c ). To confirm the promotion of osteoclastogenesis by SOV-treated osteoblasts, we evaluated the expression levels of mOC marker genes: Ctsk , Acp5 , and Atp6v0d2 . The expression levels of all mOC marker genes were significantly higher in BMMs co-cultured with total SOV-treated osteoblasts than in BMMs co-cultured with PBS-treated osteoblasts (Supplementary Fig. S3a ). Moreover, mOCs were exclusively induced on the nodules created by total SOV-treated osteoblasts in this co-culture system (Fig. 3b ), indicating that SOVs serve as a local regulator of osteoclastogenesis by regulating osteoblasts. To exclude the direct effect of SOVs on BMMs, we cultured BMMs with SOVs in the presence or absence of macrophage colony-stimulating factor (M-CSF) without osteoblasts. At 3 and 7 days after SOV treatment, we evaluated osteoclast differentiation by TRAP staining. Both PBS-treated and SOV-treated BMMs did not differentiate into mOCs within 3 or 7 days, irrespective of the presence of M-CSF (Supplementary Fig. S3b ). Therefore, we concluded that SOVs do not independently affect osteoclastogenesis. Fig. 3: SOV-F2-treated osteoblasts induce osteoclastogenesis. a Rankl and Opg mRNA levels in primary osteoblasts after treatment with PBS, total SOVs (F1 + F2), or SOV-F1 ( n = 3 biological replicates per group). b Representative image of TRAP-stained osteoclasts among BMMs co-cultured with PBS-treated osteoblasts (upper) or total SOV-treated osteoblasts (lower) ( n = 8 independent experiments per group). Dotted lines at right represent nodules created by osteoblasts. Scale bar: 100 µm. c Number of osteoclasts among BMMs co-cultured with PBS-treated osteoblasts or total SOV-treated osteoblasts per well ( n = 8 independent experiments per group). TRAP-positive multinucleated cells were counted as osteoclasts. d Representative in vivo images of calvaria from Col2.3-ECFP/TRAP-tdTomato mice of at least three independent experiments. Cyan: mature osteoblasts (mOBs) or SOVs; Red: mature osteoclasts (mOCs). Yellow circles show SOVs. mOCs were in the vicinity of mOBs secreting SOVs. Scale bar: 20 µm. e Percentages of areas where TRAP-positive cells overlapped with mOBs ( n = 5 biological replicates per group). SOV(−): fields without SOVs; SOV(+): fields with SOVs. f Transplantation model of calvarial defects. Artificial bone defects on both sides of mouse calvaria were treated with hydrogels impregnated with PBS or total SOVs. g Representative micro-CT image of calvarial defects at 8 weeks after treatment with PBS or total SOVs. Scale bar: 1000 µm ( n = 3 biological replicates per group). h Remaining calvaria defect areas at 8 weeks after treatment with PBS or total SOVs. Each point is the average area of two defects in each group ( n = 3 biological replicates per group). Data are means ± SEMs. Statistical significance was determined by one-way ANOVA with Dunnett’s multiple comparison post hoc test in ( a ), two-tailed Welch’s t -test in ( c ), and two-tailed paired t -test in ( e , h ). Full size image In the bone tissues of Col2.3-ECFP/TRAP-tdTomato mice, in which mOBs and mOCs were labeled with ECFP and tdTomato, respectively [19] , intravital imaging revealed that TRAP-positive mOCs were preferentially present in close vicinity of ECFP-positive mOBs actively secreting SOVs (Fig. 3d ). Quantitative microscopic analysis showed that TRAP-positive mOCs coincided with mOBs surrounded by SOVs (Fig. 3e ). These results suggest that SOV-treated osteoblasts stimulate osteoclast differentiation. Because SOVs inhibited osteoblast differentiation and SOV-treated osteoblasts promoted osteoclastogenesis, we evaluated the effects of SOVs on bone formation in vivo. We established bilateral calvarial defects in wild-type (WT) mice. Bone defects were exposed to hydrogels impregnated with PBS or total SOVs for 8 weeks (Fig. 3f ). The affected areas were significantly larger in the SOV-treated group than in the PBS-treated group (Fig. 3g, h ), indicating that SOVs inhibited bone repair in vivo. SOV-derived miR-143-3p suppress osteoblast differentiation by targeting Cbfb mRNA To identify the mechanism by which SOVs suppress osteoblast differentiation, we analyzed miRNAs commonly found in SOVs [21] , [22] via next-generation sequencing. We identified miR-21a-5p, miR-143-3p, and miR-148a-3p as miRNAs enriched in SOVs (Fig. 4a ). To determine the roles of these miRNAs in osteoblast differentiation, we transfected MC3T3-E1 cells with miRNA mimics and analyzed the expression levels of the osteoblastic genes Runx2 and Sp7 . The miR-143-3p mimics significantly suppressed the expression of Runx2 and Sp7 (Fig. 4b ); they also inhibited ALP activity (Fig. 4c ). The effects of miR-143-3p mimics on osteoblast differentiation were similar to the effects of total SOVs. Furthermore, transfection of miR-143-3p mimics significantly increased the expression of Rankl and suppressed the expression of Opg in MC3T3-E1 cells, consistent with the effects of SOV-treated osteoblasts on osteoclastogenesis (Supplementary Fig. S4a, b ). Fig. 4: SOV-derived miR-143-3p inhibits osteoblast differentiation by targeting Cbfb mRNA. a Next-generation sequencing-mediated miRNA profiling of SOVs. Top-ranked expression values of miRNAs in SOVs from primary osteoblasts of 10 Col2.3-ECFP mice. b Runx2 and Sp7 mRNA levels in MC3T3-E1 cells transfected with scrambled, miR-21a-5p, miR-143-3p, or miR-148a-3p mimics (The Runx2 expression in miR-21a-5p and miR-143-3p groups: n = 3; the Runx2 expression in a miR-148a-3p group and the Sp7 expression in a miR-21a-5p group: n = 4; the Sp7 expression in a miR-148a-3p group: n = 5; the Sp7 expression in a miR-143-3p group: n = 6 independent experiments, respectively). c Representative images of ALP activity in MC3T3-E1 cells transfected with scrambled, miR-21a-5p, miR-143-3p, or miR-148a-3p mimics. Scale bar: 10 mm. d Cbfb , Runx2 , and Sp7 mRNA levels in MC3T3-E1 cells transfected with siRNA negative control or Cbfb siRNA. siNCN: siRNA negative control; si Cbfb : Cbfb siRNA ( n = 4 independent experiments). The exact p value of the Cbfb expressioin: 2.34811 −9 . e Cbfb 3′ UTR constructs cloned into luciferase reporter vectors. WT 3′ UTR: wild-type sequence of the Cbfb 3′ UTR; miR-143-3p: miR-143-3p sequence; Mut 3′ UTR: mutant sequence of the Cbfb 3′ UTR. f Percentages of luciferase activity. Mut-miR143: mutated Cbfb construct with miR-143-3p mimics; WT-miR143: WT Cbfb construct with miR-143-3p mimics ( n = 4 independent experiments). g Cbfb mRNA levels in MC3T3-E1 cells treated with scrambled control or miR-143-3p mimics. Control: scrambled controls; miR-143: miR-143-3p mimics ( n = 3 independent experiments). h Cbfb mRNA levels in primary osteoblasts treated with PBS, total SOVs (F1 + F2), or SOV-F1 ( n = 6 biological replicates per group). Data are means ± SEMs. Statistical significance was determined by two-tailed paired t -test in ( b , d , f , g ) and by one-way ANOVA with Dunnett’s multiple comparison post hoc test in ( h ). Full size image To determine the molecular mechanisms by which miR-143-3p controls the expression levels of Runx2 , Sp7 , and Rankl , we analyzed its potential targets using Target Scan 7.2 and miRbase 22.1. Among hundreds of predicted mRNA targets, we focused on core-binding factor β ( Cbfb ), which may regulate the expression levels of Runx2 and Sp7 . Cbfb has been reported to form heterodimers with Runx proteins, thereby enhancing their DNA-binding capacity [30] . Osteoblast-specific Cbfb conditional deletion in Col1a1 -cre mice has also been reported to downregulate Runx2 and Sp7 , while inhibiting osteoblast differentiation [31] , [32] , [33] . Consistent with previous findings, Cbfb silencing in MC3T3-E1 cells significantly decreased the Runx2 and Sp7 mRNA levels (Fig. 4d ). To assess the ability of miR-143-3p to directly bind to Cbfb mRNA, we generated luciferase reporter constructs containing WT or mutant Cbfb mRNA binding sites (Fig. 4e ). Each construct was transfected into MC3T3-E1 cells in combination with miR-143-3p mimics. The miR-143-3p mimics significantly inhibited luciferase activity in MC3T3-E1 cells expressing the WT Cbfb binding site, but they did not inhibit luciferase activity in cells expressing the mutant binding site (Fig. 4f ). Furthermore, the expression level of Cbfb was significantly decreased in MC3T3-E1 cells transfected with miR-143-3p mimics (Fig. 4g ). These findings suggest that miR-143-3p binds directly to Cbfb mRNA. miR-143-3p drives osteoblast differentiation by targeting histone deacetylase 7 ( Hdac7 ) [34] . Therefore, we performed a luciferase assay to evaluate the ability of miR-143-3p to bind to Hdac7 mRNA. miR-143-3p mimics did not affect luciferase activity in MC3T3-E1 cells expressing WT or mutant Hdac7 binding sites (Supplementary Fig. S4c, d ). Total SOVs (F1 + F2), but not SOV-F1, significantly decreased the mRNA level of Cbfb in primary osteoblasts (Fig. 4h ). In contrast, neither total SOVs nor SOV-F1 affected Hdac7 expression (Supplementary Fig. S4e ), indicating that miR143 in SOVs does not affect the expression level of Hdac7 in SOV-treated osteoblasts. Collectively, these findings suggest that SOV-derived miR-143-3p suppresses osteoblast differentiation by targeting Cbfb . To confirm the transfer of miR-143-3p enclosed in SOVs to recipient osteoblasts, we visualized miR-143-3p in SOVs. We labeled endogenous miR-143-3p by transfecting Alexa555-conjugated miR-143-3p inhibitor into EGFP-expressing MC3T3-E1 cells and collected SOVs from the transfected cells. These SOVs were administered to non-labeled MC3T3-E1 cells and observed by confocal microscopy. Alexa555-labeled miR-143-3p colocalized with EGFP-positive vesicles in non-labeled MC3T3-E1 cells (Supplementary Fig. S4f ). This finding suggests that miR-143-3p is enclosed in SOVs and transferred into recipient cells. miR-143/145 conditional knockout increases bone mass and promotes bone mineralization in mice To further investigate the role of miR-143-3p in bone metabolism in vivo, we generated an osteoblast-specific miR-143/145 knockout (KO) mouse model (miR-143/145 Osx −/− ) by crossing miR-143/145 flox/flox mice with Osx1-Cre mice, in which Cre expression is regulated by the Osterix promoter. Because miR-143 and miR-145 are on the same gene locus, the miR-143 and -145 genes were floxed in these mice. Osx-expressing cells during the perinatal period give rise to osteoblasts, stromal cells, adipocytes, and perivascular cells; in the postnatal period, the expression of Osterix is restricted to osteoblasts [35] . In Osx1-Cre mice, Cre-mediated recombination was under the control of doxycycline. Using this system, we generated miR-143/145 Osx −/− mice expressing Cre exclusively at the postnatal period when mated to floxed-transgenic strains. Compared with control 9-week-old mice, miR-143/145 Osx −/− mice expressed low levels of miR-143-3p in primary osteoblasts (Supplementary Fig. S5a ). The mRNA levels of Runx2 , Sp7 , and Bglap in primary osteoblasts were significantly higher in miR-143/145 Osx −/− mice than in littermate control mice (Supplementary Fig. S5b ). Micro-computed tomography (CT) analyses revealed that, compared with control mice, miR-143/145 Osx −/− mice had an increased bone volume/tissue volume (BV/TV) and bone mineral density (BMD) (Fig. 5a, b ). Similarly, bone morphometric analyses showed that the parameters of bone formation—including osteoid volume/bone volume (OV/BV), mineral apposition rate (MAR), and bone formation rate/tissue volume (BFR/TV)—were significantly increased in miR-143/145 Osx −/− mice, compared with littermate control mice (Fig. 5c, d ). Although the osteoblast surface/bone surface (Ob.S/BS) was comparable between miR-143/145 Osx −/− and control mice (Supplementary Fig. S5c ), the cuboidal Ob.S/Ob.S (ratio of Ob.S of mOBs to Ob.S of total osteoblasts) was significantly higher in miR-143/145 Osx −/− mice than in control mice (Fig. 5d ). Therefore, osteoblast-specific miR-143/145 depletion increased bone mass and promoted mineralization. Fig. 5: miR-143/145 conditional KO increases bone mass and promotes mineralization in mice. a Representative micro-CT images of the femurs of 9-week-old control ( n = 4 biological replicates) and osteoblast-specific miR-143/145 KO (miR-143/145 Osx −/− ) mice ( n = 5 biological replicates). Scale bars: 1000 μm. b Micro-CT-based assessment of metaphyseal regions of distal femurs of 9-week-old control ( n = 4 biological replicates) and miR-143/145 Osx −/− ( n = 5 biological replicates) mice. BV: bone volume; TV: tissue volume; BMD: bone mineral density. c , d Bone morphometric analysis of metaphyseal regions of distal femurs of 9-week-old control and miR-143/145 Osx −/− mice ( n = 3 biological replicates per group). Calcein double signals in a representative femur section from a control or miR-143/145 Osx −/− mouse on cortical surfaces and magnified view (inset). Scale bars: 100 µm ( c ). Bone formation parameters ( d ). OV: osteoid volume; MAR: mineral apposition rate; BFR: bone formation rate; Ob.S: osteoblast surface. e Transplantation model of calvarial defects. Artificial bilateral defects on mouse calvaria were treated with total SOVs from miR-143/145 KO or WT mice. f Representative micro-CT image of calvarial defects at 2 weeks after treatment with SOVs from miR-143/145 KO or WT mice ( n = 3 biological replicates per group). Scale bar: 2000 µm. g Remaining defect areas. miR-143/145 KO: mice treated with total SOVs from miR-143/145 KO mice; WT: mice treated with SOVs from WT mice ( n = 3 biological replicates per group). Data are means ± SEMs. Statistical significance was determined by two-tailed unpaired t -test in ( b , d ) or by two-tailed paired t -test in ( g ). Full size image miR-143/145 conditional knockout decreases osteoclast activity after parathyroid hormone administration in vivo Because deletion of miR143-3p in osteoblasts in vivo using miR-143/145 Osx −/− mice did not influence any parameters of osteoclast formation or function (Supplementary Fig. S5c ), we performed bone morphometric analyses of miR-143/145 Osx −/− mice under the high bone-metabolic turnover condition. We intermittently injected parathyroid hormone (PTH) into WT and miR-143/145 Osx −/− mice, then performed micro-CT analysis, bone morphometric analysis, and measurement of the urine C-terminal telopeptide-1 (CTX-1) level, which reflects osteoclast activity [36] . Micro-CT and bone morphometric analyses revealed that there were no significant differences in BV/TV between PTH-treated WT mice and PTH-treated miR-143/145 Osx −/− mice (Supplementary Fig. S6a, c ). The urine CTX-1 level (corrected for urine creatinine) was significantly lower in miR-143/145 Osx −/− mice than in WT mice (Supplementary Fig. S6b ). Consistent with those findings, morphometric analyses revealed that eroded surface/bone surface (ES/BS), osteoclast number/bone surface (N.Oc/BS), and osteoclast surface/bone surface (Oc.S/BS) were significantly lower in PTH-treated miR-143/145 Osx −/− mice than in PTH-treated WT mice (Supplementary Fig. S6c ). Therefore, miR-143/145 osteoblast-specific knockout mice showed significantly decreased osteoclast activity and number compared with WT mice, indicating that miR-143/145 in osteoblasts promotes osteoclastogenesis in vivo under a high bone-metabolic turnover condition (Supplementary Fig. S6b, c ). MiR-143/145-deleted SOVs reversed the inhibition by SOVs of bone repair To investigate the effects of miR-143 in SOVs on osteoblast differentiation and osteoclastogenesis, we analyzed the effects of SOVs from miR-143/145 Osx −/− mice on Runx2 , Sp7 , and Rankl expression levels in osteoblasts in vitro. The miR-143/145-deleted SOVs significantly reversed the inhibition (by WT SOVs) of Runx2 and Sp7 expression (Supplementary Fig. S7a ). In addition, miR-143/145-deleted SOVs significantly reversed the enhancing effect of WT SOVs on Rankl expression in osteoblasts (Supplementary Fig. S7b ). Next, to analyze the function of miR-143 in SOV on bone formation in vivo, bilateral calvarial defects in WT mice were exposed to gelatin hydrogels impregnated with total SOVs from miR-143/145 KO or WT mice (Fig. 5e ). At 2 weeks after the procedure, the affected areas were significantly smaller in areas treated with total SOVs from miR-143/145 KO mice, than in areas treated with total SOVs from WT mice (Fig. 5f, g ), suggesting that miR-143 in SOVs impairs bone repair. In summary, these results suggest that SOVs inhibit osteoblastic bone formation and stimulate osteoclast formation through an miR-143-mediated mechanism, which promotes reciprocal reserve phase switch (Fig. 6 ). Fig. 6: Graphical abstract of the role of small osteoblast vesicles in bone remodeling. Interactions among mOBs via SOVs inhibit osteoblastic bone formation and stimulate osteoclast formation, thus switching from the bone formation phase to the bone resorption phase. Full size image Bone formation by osteoblasts is a long-lasting phase that may last several months and is tightly regulated during bone remodeling [37] . Although the signaling and transcriptional regulation of osteoblast differentiation have been investigated [38] , [39] , the terminating factors of bone formation and initiating factors of subsequent bone resorption remain elusive. Using an intravital bone imaging approach, we identified intercellular communication among osteoblasts via SOVs and demonstrated negative regulation of bone formation and positive regulation of bone resorption by SOVs derived from mOBs. Osteoblasts co-cultured with SOVs inhibited osteoblastogenesis and enhanced the osteoclastogenesis of BMMs. The effect of SOVs on osteoclastogenesis was not a direct effect of SOVs on BMMs; it was caused by phenotypic changes, such as the upregulation of Rankl in SOV-treated osteoblasts. Consistent with this finding, mOCs were exclusively induced on nodules that had been created by total SOV-treated osteoblasts in the co-culture system, indicating that osteoblast–osteoblast communication via SOVs is important for spatiotemporal regulation of osteoclastogenesis. These observations suggest that communication among osteoblasts by means of SOVs induces a phase transition from bone formation to bone resorption as a spatiotemporal bone remodeling regulation mechanism. It is widely accepted that bone formation follows bone resorption [2] ; however, our findings suggest that osteoblast–osteoblast communication via SOVs can directly induce osteoclastogenesis, providing further insights into bone homeostasis. The possibility of immediate transition to bone resorption after the bone formation phase without a resting phase remains controversial [6] . We believe that direct transition from bone formation to bone resorption may happen under high turnover conditions and dysregulated remodeling conditions, such as osteoporosis [40] , [41] and bone repair. Future studies are needed to confirm this hypothesis. We identified Cbfb mRNA as a target of miR-143-3p in osteoblasts. The bone phenotype of miR-143/145 Osx −/− mice was consistent with the phenotype of Cbfb conditional KO ( Cbfb col1a1 −/− ) mice [33] . Cbfb col1a1 −/− mice in the postnatal period exhibited reduced bone mass, MAR, and Runx2 expression. Although the number of osteoblasts was unchanged, the number of active osteoblasts decreased in Cbfb col1a1 −/− mice [33] . Notably, miR-143/145 Osx −/− mice exhibited a phenotype opposite to the findings in Cbfb col1a1 −/− mice (i.e., increased bone mass, MAR, Runx2 mRNA expression, and ratio of mOBs to total osteoblast area [cuboidal Ob.S/Ob.S]). MiR-143 was previously shown to inhibit Sp7 mRNA expression in osteoblasts, as indicated by luciferase assay results using human Sp7 mRNA sequences [42] , [43] . However, according to two major databases, Target Scan 7.2 and miRBase 22.1, murine Sp7 mRNA does not have complementary base sequences to bind to mmu-miR-143-3p. Thus, the suppressed Sp7 expression in murine osteoblasts transfected with miR-143-3p mimics was presumably not caused by direct binding of miR-143-3p mimics to Sp7 mRNA; it was likely dependent on the decreased expression of Runx2 caused by miR-143-3p binding to Cbfb mRNA. In addition to the effect of miR-143-3p on osteoblast differentiation, we demonstrated that miR-143-3p increased the Rankl/Opg ratio in MC3T3-E1 cells. Although increasing Rankl/Opg in osteoblasts should enhance osteoclastogenesis, the parameters of osteoclast formation and function were not affected in miR-143/145 Osx −/− mice at steady state (Supplementary Fig. S5c ), consistent with the phenotype of Cbfb col1a1 −/− mice [33] . However, the parameters were significantly decreased in miR-143/145 Osx −/− , compared with control mice, following intermittent PTH administration. The phenotypes of osteoclast formation and function in miR-143/145 Osx −/− mice were enhanced by intermittent PTH administration with increasing bone turnover. In addition to endogenous effects in osteoblasts, we evaluated the effects of miR-143 in SOVs. MiR-143-containing SOVs significantly upregulated Rankl expression in SOV-treated osteoblasts; this change was reversed by miR-143/145-deleted SOVs. This finding suggests that miR-143-3p in SOVs induced a phenotypic change of osteoblasts to enhance osteoclastogenesis. Therefore, miR-143 is essential for the ability of SOVs to inhibit bone formation and promote bone resorption. Although miR-143 directly binds to Cbfb mRNA and inhibits osteoblast differentiation, the mechanism by which miR-143 increases Rankl expression in osteoblasts is unknown. Runx2 regulates Rankl expression by condensing the chromatin structure at the Rankl enhancer and promoter regions in a histone deacetylase 3-dependent manner [44] . Decreased Runx2 expression might have led to Rankl upregulation in osteoblasts treated with SOVs or miR-143-3p mimics. However, the miR-143/145-deleted SOVs did not totally cancel the effect of WT SOVs on Runx2 and Rankl expression, implicating other factors in SOVs. Other proteins and nucleic acids in SOVs may also affect osteoblast differentiation and function. Future studies are needed to identify functional proteins and/or other components in these vesicles. In conclusion, our findings provide an insight into the in vivo interactions among mOBs via SOVs and demonstrate that SOVs are critical factors regulating reciprocal reversal switch in a miR-143-dependent mechanism. Mouse model C57BL/6J mice were obtained from CLEA Japan (Tokyo, Japan). The generation of Col1a1*2.3-ECFP and TRAP-tdTomato transgenic mice was described previously [18] , [19] . miR-143/145-floxed mice and miR-143/145 KO mice [45] were kindly provided by Thomas Boettger and Thomas Braun, Max-Plank-Institute, Germany. To generate the loxP-mice, we generated a miR-143/145 lox/lox targeting vector by subcloning the miR-143/145 locus [45] . A loxP site was inserted into the HindIII site 1 kb upstream of miR-143, and a second loxP site plus a neomycin resistance cassette was inserted into the HindIII site 2.3 kb downstream of miR-145. Mice were generated as described previously [45] . Osx1-GFP:Cre mice were obtained from the Jackson Laboratory (Stock Number: 006361). miR-143/145 Osx −/− mice and their littermates were fed a diet containing doxycycline 0.02% (v/v) via breastfeeding until becoming 4 weeks old. Nine-week-old mice were analyzed for bone phenotypic changes. Male mice (10–20 weeks of age) were used unless indicated otherwise. The number of animals used is indicated in the corresponding figure legend. All mice were housed in specific pathogen-free facilities under a 12 h light/dark cycle and controlled temperature (19–23 °C) and humidity (55 ± 10%). Mice were given standard laboratory chow diet and water ad libitum unless indicated otherwise. Animal studies were approved by the Institutional Review Board of Osaka University. Cell culture In vitro osteoblast differentiation has been described previously [19] , [46] . Briefly, bone marrow cells (5.3 × 10 5 per cm 2 ) were collected by flushing long bones of mice and maintained for 3 days in α-minimum essential medium (α-MEM) containing 10% fetal bovine serum (FBS) and 1% penicillin–streptomycin at 37 °C in a humidified incubator containing 5% CO 2 . The cells were maintained in osteogenic medium (α-MEM, 10% FBS, 1% penicillin–streptomycin, 50 mg/mL ascorbic acid, and 10 mM beta-glycerophosphate) for 14 days to promote osteoblastic differentiation and mineralization. The osteogenic medium was refreshed every 3 days. MC3T3-E1, a clonal osteoblastic cell line derived from newborn mouse calvaria, was purchased from the American Type Culture Collection (CRL-2593™: ATCC, Manassas, VA, USA). Cells (1.05 × 10 4 per cm 2 ) were maintained for 2 days in α-MEM containing 10% FBS and 1% penicillin–streptomycin. For osteoblastic differentiation and mineralization, cells were maintained in osteogenic medium, which was refreshed every 3 days. To generate BMMs, non-adherent bone marrow cells from C57BL/6J mice were seeded in a 10 cm Petri dish and cultured in α-MEM containing 10% FBS, 1% penicillin–streptomycin, and 10 ng/mL M-CSF. After 3 days, adherent cells were collected in enzyme-free cell dissociation buffer (Millipore, Burlington, MA, USA) at 37 °C and used as BMMs. Intravital multiphoton imaging Col1a1*2.3-ECFP mice and Col2.3-ECFP/TRAP-tdTomato double transgenic reporter mice were anesthetized with isoflurane (Escain; 2.5% vaporized in an 80:20 mixture of O 2 and air), and the hair on the neck and the scalp was removed using hair removal lotion (Epilat). The front-parietal skull was exposed after the skin incision, and the head was immobilized in a custom-made stereotactic holder [19] . Intravital multiphoton imaging was performed as described previously [15] , [16] , [17] , [18] , [19] . The imaging system for Col1a1*2.3-ECFP mice was composed of a multiphoton microscope (LSM 780 NLO; Carl Zeiss) driven by a laser (Chameleon Vision II Ti: Sapphire; Coherent) at 860 nm and an upright microscope equipped with a 20× water immersion objective (W Plan-APOCHROMAT; Carl Zeiss). The microscope was enclosed in an optimally customized chamber in which the temperature was controlled to warm the anesthetized mice. The heart rate of the mice was monitored by electrocardiography. Fluorescent cells were detected by a spectral imaging microscope. The step size was adjusted to 2 μm to create Z-stack images; five slices were captured as the depth was 10 µm. Images were recorded with pixel dimensions of 0.26 μm and a time interval of 5 min. Raw imaging data were processed to 3D images and maximum intensity projection (MIP) on Z with NIS Elements software (Nikon). Constant g corrections were applied to all images (g = 0.65) with NIS Elements software to enhance the signal-to-noise ratio. MIP data were edited to surface images with Imaris software (Bitplane). The tracking analysis was performed using the surface function. Surface objects were created manually and filtered according to tracking time (>20 min). The imaging system for Col2.3-ECFP/TRAP-tdTomato mice consisted of an upright multiphoton microscope (A1R MP+; Nikon) with a 25× water immersion objective (CFI75 Apo 25XC W 1300; Nikon). The system was driven by lasers (Chameleon Vision II Ti: Sapphire; Coherent, Inc.); the main laser was tuned to 860 nm to detect ECFP and second harmonic generation, and the sub-laser was tuned to 1040 nm to detect tdTomato. Multi-fluorescence images were acquired under a Nikon upright microscope using four external non-descanned detectors equipped with dichroic and emission filters, including an infrared-cut filter (DM685), three dichroic mirrors (DM458, DM506, and DM605), and three emission filters (417/60 for the second harmonic generation image, 480/40 for ECFP, 583/22 for tdTomato). In vitro time-lapse imaging Primary osteoblasts from Col2.3-ECFP mice cultured for 10–14 days and CD63-GFP MC3T3-E1 cells cultured for 3 days were observed, and time-lapse images were captured using a Nikon A1-Si confocal laser scanning microscope. Primary osteoblasts and CD63-GFP MC3T3-E1 cells were excited at 457 nm and 561 nm for primary osteoblasts and 488 nm for CD63-GFP MC3T3-E1 cells (Coherent). Autofluorescence was collected with photomultiplier-type detectors at wavelength emission windows of 482/35 nm for the 457 nm laser to detect ECFP, 525/50 nm for the 488 nm laser to detect EGFP, and 595/50 nm for the 561 nm laser to detect PKH26. Images were recorded with pixel dimensions of 0.31 or 0.63 µm. Raw imaging data were edited with NIS Elements software (Nikon). Constant g corrections were applied to all images (g = 0.65) to enhance the signal-to-noise ratio. MIP data were edited to surface images with Imaris software (Bitplane). Isolation of SOVs SOVs were isolated from primary osteoblasts or MC3T3-E1 cells according to a previously described procedure [47] . Briefly, the culture medium was replaced with EV-free osteogenic medium (containing 10% EV-free FBS prepared by centrifugation at 70,000 × g overnight instead of 10% FBS) 2 days before SOV collection. The culture medium was collected, and cells were treated with 0.2% collagenase P (Roche) for 1 h at 37 °C followed by 0.25% trypsin (containing 0.02% EDTA) for 10 min at 37 °C. The culture medium and digested cells were centrifuged at 300 × g for 5 min at 4 °C to separate cells, and the supernatant was centrifuged at 2000 × g for 20 min at 4 °C to remove debris. The supernatant was further centrifuged at 16,500 × g for 20 min at 4 °C. The pellet containing SOVs was resuspended in PBS and divided into two groups: total SOVs (F1 + F2) and SOV-F1 (0.22-µm filtration). Both groups were treated with 0.5 mg/mL RNase A (Nippon Gene) at 37 °C for 20 min and were centrifuged at 16,500 × g for 20 min to wash. For proteinase K treatment, SOVs were treated with proteinase K (final concentration: 0.1 mg/mL) for 20 min at 37 °C, then incubated for 5 min at 90 °C to inactivate proteinase K. EV experiments were performed based on the criteria presented by the International Society of Extracellular Vesicles position paper in 2018 [26] . PKH-labeling of SOVs SOVs were collected from primary osteoblasts cultured for 14 days. SOVs were then labeled with PKH26 Red Fluorescent Cell Linker Kit (Sigma-Aldrich) at room temperature for 5 min, blocked with FBS, and washed four times with PBS in accordance with the manufacturer’s instructions. Primary osteoblasts cultured for 10–14 days were treated with PKH-labeled SOVs and were observed under a confocal microscope. Generation of stable cell lines The lentiviral vector pCT-CD63-GFP (System Biosciences) and a packaging plasmid for generation of a CD-63-GFP MC3T3-E1 cell line or the pMYs-IRES-GFP Retroviral Vector (CELL BIOLABS) for generation of a MC3T3-E1 GFP cell line were transfected into HEK293T cells using PEI max (Polysciences). MC3T3-E1 cells were transduced with virus-containing medium from transfected HEK293T cells and polybrene (Merck) 48 h after transfection. Transduced MC3T3-E1 cells expressing GFP were selected using a cell sorter (SONY), and single cells were cultured to establish a cell line. Imaging flow cytometry Primary osteoblast samples from Col1a1*2.3-ECFP transgenic mice were prepared after 14 days of culture and were treated with PKH-labeled total SOVs. Samples were then analyzed using an ImageStreamX Mark II cytometer (Amnis, EMD Millipore) at a low flow rate and high sensitivity using 60-fold magnification. Cells were collected by centrifugation at 300 × g after treatment with 0.2% collagenase P (Roche) for 1 h at 37 °C, followed by 0.25% trypsin (containing 0.02% EDTA) for 10 min. Single-cell suspensions (2 × 10 7 /mL) in flow cytometry (FACS) buffer were incubated with PE-Cy7 conjugated anti-mouse CD45 antibody (BioLegend) diluted in FACS buffer at 1:100 ratio for 15 min. CFP, CD45-PE-Cy7, and PKH26 were excited at 495 nm (CFP) and 488 nm (CD45-PECy7 and PKH26) and were detected at 435–505 nm (CFP), 745–785 nm (CD45-PECy7), and 642–745 nm (PKH26). Flow cytometric data were analyzed using IDEAS software (Amnis, EMD Millipore). Transmission electron microscopy Collected total SOVs (F1 + F2) or SOV-F1 were fixed with iPGell (Geno Staff). Samples were washed and post-fixed in 1% osmium tetroxide at 4 °C for 90 min. Subsequently, samples were dehydrated in graded ethanol with propylene oxide and embedded in epoxy resin. Semi-thin sections (75 nm) were mounted on copper grids and observed using an H-7650 transmission electron microscope (Hitachi Electronic Instruments). Nanoparticle tracking analysis Nanoparticle tracking analysis was performed using Nanosight LM10 and NTA2.3 software (NanoSight). Samples were diluted 100-fold with PBS, and 30-s videos were recorded at the same camera level and detection threshold on the same day. The temperature was monitored throughout the measurements. Treatment of SOVs Primary osteoblasts cultured in 24-well plates for 6 days were treated with PBS, total SOVs (F1 + F2), or SOV-F1. SOVs were collected from primary osteoblasts that had been cultured for 14 days. The final concentrations of total SOVs (F1 + F2) and SOV-F1 were 1–5 × 10 9 /mL. MC3T3-E1 cells cultured in 24-well plates for 21 days were treated with PBS, total SOVs (F1 + F2), or SOV-F1. SOVs were collected from MC3T3-E1 cells that had been cultured for 28 days. The final concentrations of total SOVs (F1 + F2) and SOV-F1 were 1–5 × 10 9 /mL. Total RNAs were extracted 2 days after treatment, and ALP staining was performed 5 days after treatment. For collagen and Alizarin Red S staining, we treated primary osteoblasts cultured in 24-well plates for 3 days with PBS, total SOVs (F1 + F2), or SOV-F1 from primary osteoblasts that had been cultured for 14 days, then stained them 3 days after treatment. RNA isolation and quantitative real-time PCR Total RNA and cDNA were prepared using the Maxwell 16 LEV RNA purification kit (Promega) and Superscript III reverse transcriptase (Thermo Fisher Scientific) in accordance with the manufacturer’s instructions. Quantitative real-time PCR (qPCR) was performed using a TP800 Dice Real-Time Thermal Cycler System (TaKaRa). Gene expression was calculated relative to that of the housekeeping gene β-actin. 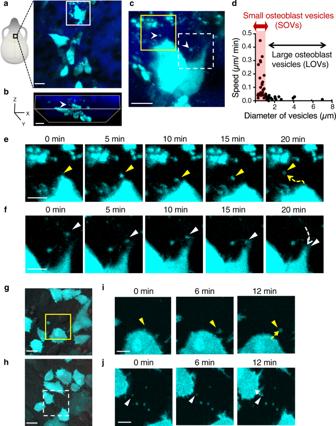Fig. 1: Communication among osteoblasts via small osteoblast vesicles in vivo and in vitro. aSchematic representation of mouse skull bone (left) and an intravital multiphoton, maximum-intensity projection image of skull bone tissues from Col2.3-ECFP mice (a representative image, at least three independent experiments) (right). Cyan: mature osteoblasts (mOBs) and extracellular vesicles (EVs) from mOBs; blue: bone surface, second harmonic generation. Scale bar: 20 μm.bThree-dimensional image of visual field shown in (a). Arrowhead indicates an EV. Scale bar: 20 μm.cMagnified view of region outlined in (a). Arrowheads indicate EVs. Scale bar: 10 μm.dSpeed of mOB-derived EVs by tracking analysis of EVs shown in (c) (n= 51). SOVs: small osteoblast vesicles with a diameter of ≤1 µm; LOVs: large osteoblast vesicles with a diameter of >1 µm.eConsecutive time-lapse images of SOVs released by mOBs indicated by yellow lines in (c). Arrowheads and dotted lines indicate SOVs and their tracks, respectively. Scale bar: 5 µm.fConsecutive time-lapse images of SOVs taken up by mOBs indicated by dotted lines in (c). Arrowheads and dotted lines indicate SOVs and their tracks, respectively. Scale bar: 5 µm.g,hRepresentative images of primary osteoblasts of Col2.3-ECFP mice of at least three independent experiments. Cyan: mOBs and mOB-derived EVs. Scale bar: 20 µm.iConsecutive time-lapse images of released SOVs indicated by yellow lines in (g). Arrowheads and dotted lines indicate SOVs and their tracks, respectively. Scale bar: 10 µm.jConsecutive time-lapse images of internalized SOVs indicated by dotted lines in (h). Arrowheads and dotted lines indicate SOVs and their tracks, respectively. Scale bar: 10 µm. The primer sequences used are listed in Supplementary Table 1 . ALP and TRAP staining ALP substrate solution was prepared by dissolving 0.006% (w/v) Naphthol AS-MX phosphate (Sigma-Aldrich) in 0.1 M Tris (pH 8.0) and adding 0.1% (w/v) Fast blue BB salt (Sigma-Aldrich). After fixation in 4% paraformaldehyde, cells were stained with ALP substrate solution for 10 min at room temperature in the dark and were rinsed with distilled water. For quantitative analyses, ALP activities were assessed using a TRACP & ALP Assay Kit (TaKaRa Bio) in accordance with the manufacturer’s instructions. Cells were washed with saline and were lysed using a commercial lysis solution. Samples were treated with ALP substrate for 15 min at 37 °C, and the absorbance at 405 nm was measured using a microplate reader. TRAP substrate solution was prepared by dissolving 0.01% (w/v) Naphthol AS-MX phosphate (Sigma-Aldrich) in TRAP buffer (pH 5.0, 66 mM sodium acetate and 45 mM sodium tartrate) supplemented with 0.06% (w/v) Fast Red Violet LB salt (Sigma-Aldrich). After fixation in 4% paraformaldehyde, cells were permeabilized with acetone ethanol (1:1) solution and stained with TRAP substrate solution for 5 min at room temperature. Collagen staining and Alizarin Red S staining For collagen staining, after fixation in Kahle Fixative, cells were stained with a dye solution in accordance with the manufacturer’s instructions (Chondex). For Alizarin Red S staining, after fixation in 4% paraformaldehyde cells were stained with 2% Alizarin Red S solution (Fujifilm Wako Pure Chemical Corporation). Cell death analysis Primary osteoblasts cultured for 6 days were treated with PBS, total SOVs (F1 + F2), or SOV-F1 for 6 days. Cells were analyzed using a cell sorter (SH800, Sony) to detect 7-AAD signals. Single-cell suspensions (1 × 10 6 /mL) were incubated with CD45-PECy7 (BioLegend) diluted in FACS buffer at 1:100 ratio for 15 min, and stained with 10 μg/ml 7-AAD (BD Biosciences) immediately before analysis to detect dead cells. Flow cytometry data were analyzed using FlowJo software (TreeStar). Co-culture system for osteoclastogenesis in vitro BMMs were co-cultured with total SOV-treated osteoblasts or PBS-treated osteoblasts using a modified osteoclast culture method [48] . Primary osteoblasts cultured for 6 days were treated with total SOVs or PBS. The culture medium containing SOVs or PBS was removed 2 days after treatment; BMMs (0.63 × 10 5 /cm 2 ) were co-cultured with the osteoblasts in osteogenic medium with 100 ng/mL 1 alpha,25-dihydroxyvitamin D3 (Calcitriol, Fujifilm Wako Pure Chemical Corporation). Three days later, TRAP-positive multinucleated cells were counted as mOCs after TRAP staining and qRT-PCR of mature osteoclast marker genes were performed. To evaluate the direct effect of SOVs on osteoclastogenesis, BMMs (1.5 × 10 5 /cm 2 ) were cultured for 2 days with 10 ng/mL M-CSF. SOVs (final concentration of 1–5 × 10 9 /mL) were added to the BMMs with or without 10 ng/mL M-CSF. Three and seven days later, TRAP staining was performed. miRNA isolation and qPCR Total RNA containing miRNAs was prepared using a miRNeasy Mini Kit (Qiagen). qPCR was performed using a TaqMan Advanced miRNA kit in accordance with the manufacturer’s instructions. The expression level of each miRNA was calculated relative to that of miR-423-5p. Next-generation miRNA sequencing SOV-derived RNAs from primary osteoblasts cultured for 14 days were isolated using miRNeasy Mini Kit (Qiagen). Small RNA libraries were constructed using the NEBNext Small RNA Library Prep Set for Illumina (NEB) in accordance with the manufacturer’s instructions, and libraries were sequenced on the HiSeq 2500 platform (Illumina) in 75-base pair single-end reads. The miRNA-seq analysis was conducted using CLC Genomics Workbench v9.5.3 (Qiagen) in accordance with the small RNA alignment and small RNA analysis pipeline using default parameters. Adapters were trimmed to retain only reads of length 15–25 bp. Of 1,927,614 trimmed reads, 832,524 were then mapped and annotated against the miRBase (version 21). Read counts of the annotated miRNAs were exported from the CLC Genomics Workbench. Raw data were deposited in the NCBI GEO database (GSE144512). Transfection of miRNA mimics MC3T3-E1 cells were maintained with serum- and antibiotic-free medium for 24 h. miRNA mimics of miR-143-3p, miR-21-5p, and miR-148-3p and mimic negative control (mirVana™ miRNA mimics, Thermo Fisher Scientific) were transfected into MC3T3-E1 cells using Lipofectamine RNAiMAX (Thermo Fisher Scientific). RNA was extracted 2 days after transfection. Transfection of siRNAs Cbfb siRNAs (Stealth RNAi™ siRNA, Thermo Fisher Scientific) or negative control siRNAs (Stealth RNAi™ siRNA Negative Control Lo GC, Thermo Fisher Scientific) were transfected into MC3T3-E1 cells using Lipofectamine RNAiMAX (Thermo Fisher Scientific). RNA was extracted 2 days after transfection. Luciferase reporter assay WT Cbfb or Hdac7 sequence fragments containing predicted miR-143-3p binding sites were chemically synthesized and cloned downstream of the luciferase gene in the pmirGLO Dual-Luciferase miRNA Target Expression Vector (Promega) between SacI and XbaI sites. Fragments with mutant binding sites were also synthesized and cloned as controls. MC3T3-E1 cells cultured in 96-well plates (1 × 10 4 /well) were co-transfected with the recombinant reporter plasmids and miR-143-3p mimic or scramble negative controls using Lipofectamine 2000 (Invitrogen). Cells were harvested 48 h after transfection, and luciferase activity was measured using the Dual-Glo Luciferase Assay System (Promega) and Luminescent Micro Plate Reader (Centro XS3 LB960, Berthold Technologies). Firefly luciferase activity was normalized to that of Renilla luciferase. Visualization of transfer of miR-143-3p in SOVs MC3T3-E1 EGFP cells were transfected with Alexa Fluor 555-conjugated miR-143-3p inhibitor (mirVana miRNA Inhibitor, Thermo Fisher Scientific). SOVs were collected from the transfected cells 1 day after transfection. MC3T3-E1 cells were treated with the collected SOVs, and the cells were observed with a confocal microscope (Nikon A1-Si) 1 day after treatment. Autofluorescence was collected with photomultiplier-type detectors at wavelength emission windows of 452/45 nm (for the 488 nm laser to detect EGFP) and 525/50 nm (for the 488 nm laser to detect Alexa Fluor 555). Images were recorded with pixel dimensions of 0.05 µm. The step size was adjusted to 0.1 μm to create Z-stack images; 96 slices were captured using a depth of 9.6 µm. Raw imaging data were edited using NIS Elements software (Nikon). Microstructure analysis The right femurs were extracted from 9-week-old osteoblast-specific deletion of miR-143/145 (miR-143/145 Osx −/− ) and floxed (miR-143/145 flox/+ ) male mice (body weight: 20–24 g). A cone-beam X-ray micro-CT system (ScanXmate-RB090SS150; Comscantecno) was used to obtain CT images of the distal ends of femurs. The settings were as follows: tube voltage, 70 kV; tube current, 0.1 mA; and voxel size, 12.0 µm. The 3D images were reconstructed and analyzed using TRI/3D-BON software (RATOC System Engineering). Regions of interest were drawn 50 µm from the end of each epiphyseal growth plate to points 0.5 mm along the cortical wall. Bone morphometric analysis The left femurs were extracted from 9-week-old osteoblast-specific deletion of miR-143/145 (miR-143/145 Osx −/− ) and floxed (miR-143/145 flox/+ or miR-143/145 flox/+ ) male mice and were performed bone morphometric analysis as described previously [49] . For toluidine blue staining, femurs were excised, fixed in 100% ethanol, and embedded in glycolmethacrylate. For double staining of cortical bone surfaces, mice were injected subcutaneously with calcein (8 mg/kg) at 4 days or 1 day before being sacrificed. Phenotype of osteoblast-specific deletion of miR-143/145 in vitro Primary osteoblasts from 9-week-old miR-143/145 Osx −/− and littermate floxed (miR-143/145 flox/flox ) male mice were analyzed. RNA extraction was performed 10 days after starting osteoblast differentiation. The expression of miR-143-3p in primary osteoblasts cultured for 14 days was assessed. PTH administration in vivo Intermittent PTH injections were conducted to 5-week-old female WT and miR-143/145 Osx −/− mice (PTH: human PTH (1–34) [teriparatide; Asahi Kasei Pharma Corporation]). The dose of human PTH (1–34) was 40 µg/kg body weight per day for 5 days per week, delivered via subcutaneous injection for 4 weeks, as described previously [36] . Micro-CT analysis, bone morphometric analysis, and measurement of the urine C-terminal telopeptide-1 (CTX-1) level were performed after PTH administration at 9 weeks of age (body weight 18–22 g). The right femurs were extracted for micro-CT analysis, and the left femurs were used for bone morphometric analyses with Villanueva bone staining embedded in methylmethacrylate as described above. For measurement of CTX-1, mice were fasted for 12 h before urine sampling by bladder puncture. 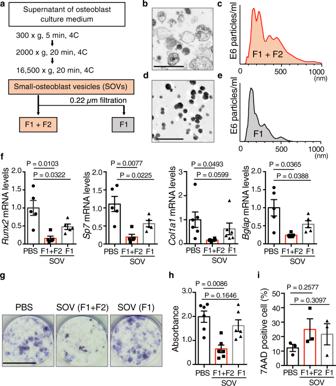Fig. 2: SOV-F2 inhibits osteoblast differentiation. aSchematic representation of SOV isolation via differential centrifugation. F1: fraction 1; F2: fraction 2.bTransmission electron micrograph of total SOVs (at least three independent fields from 1 mouse). Scale bar: 1 µm.cNanoparticle tracking analysis of total SOVs (at least three independent experiments).dTransmission electron micrograph of SOV-F1 after 0.22 µm filtration (at least three independent fields from 1 mouse). Scale bar: 500 nm.eNanoparticle tracking analysis of SOV-F1 after 0.22 µm filtration (at least three independent experiments).fRunx2,Sp7,Col1a1, andBglapmRNA levels in osteoblasts treated with PBS, total SOVs (F1 + F2), or SOV-F1 (Runx2,Sp7andBglap:n= 5;Col1a1:n= 6 biological replicates per group).g,hALP activity in osteoblasts treated with PBS, total SOVs (F1 + F2), or SOV-F1 (n= 6 biological replicates per group). Representative images (g) and quantitative analysis (h) Scale bar: 10 mm.iPercentages of 7-AAD-positive apoptotic cells among CD45-negative primary osteoblasts at 6 days after treatment with PBS, total SOVs (F1 + F2), or SOV-F1 (n= 3 biological replicates per group). Data are means ± SEMs. Statistical significance was determined by one-way ANOVA with Dunnett’s multiple comparison post hoc test (f,h,i). CTX-1 and creatinine levels in the urine samples were measured by enzyme-linked immunosorbent assay (RatLaps TM; Immunodiagnostics Systems) and enzymatic method (Wako), respectively. The CTX-1 level was corrected for the creatinine concentration. SOV transplantation on calvarial bone defects C57BL/6 J male mice were anesthetized with isoflurane, and an incision was made on the head skin to expose the calvaria. Artificial calvarial defects were created on both sides using surgical punches and needles. 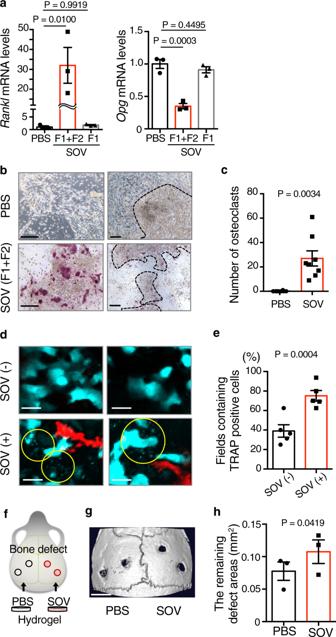Fig. 3: SOV-F2-treated osteoblasts induce osteoclastogenesis. aRanklandOpgmRNA levels in primary osteoblasts after treatment with PBS, total SOVs (F1 + F2), or SOV-F1 (n= 3 biological replicates per group).bRepresentative image of TRAP-stained osteoclasts among BMMs co-cultured with PBS-treated osteoblasts (upper) or total SOV-treated osteoblasts (lower) (n= 8 independent experiments per group). Dotted lines at right represent nodules created by osteoblasts. Scale bar: 100 µm.cNumber of osteoclasts among BMMs co-cultured with PBS-treated osteoblasts or total SOV-treated osteoblasts per well (n= 8 independent experiments per group). TRAP-positive multinucleated cells were counted as osteoclasts.dRepresentative in vivo images of calvaria from Col2.3-ECFP/TRAP-tdTomato mice of at least three independent experiments. Cyan: mature osteoblasts (mOBs) or SOVs; Red: mature osteoclasts (mOCs). Yellow circles show SOVs. mOCs were in the vicinity of mOBs secreting SOVs. Scale bar: 20 µm.ePercentages of areas where TRAP-positive cells overlapped with mOBs (n= 5 biological replicates per group). SOV(−): fields without SOVs; SOV(+): fields with SOVs.fTransplantation model of calvarial defects. Artificial bone defects on both sides of mouse calvaria were treated with hydrogels impregnated with PBS or total SOVs.gRepresentative micro-CT image of calvarial defects at 8 weeks after treatment with PBS or total SOVs. Scale bar: 1000 µm (n= 3 biological replicates per group).hRemaining calvaria defect areas at 8 weeks after treatment with PBS or total SOVs. Each point is the average area of two defects in each group (n= 3 biological replicates per group). Data are means ± SEMs. Statistical significance was determined by one-way ANOVA with Dunnett’s multiple comparisonpost hoctest in (a), two-tailed Welch’st-test in (c), and two-tailed pairedt-test in (e,h). Round defects with diameters of 1.0 mm were created for comparison between the total SOV-treated group and PBS-treated group; round defects with diameters of 1.5 mm were created for comparison of the effect of total SOVs from miR-143/145 KO mice with the effect of total SOVs from WT mice. A gelatin hydrogel sheet (MedGel II PI9, Nitta-gelatin, Japan) was cut to the same size as the defect and impregnated with PBS or SOVs (1–5 × 10 9 ). The hydrogels were transplanted into either side of the calvaria defect. A micro-CT assessment was performed after 8 weeks (for the PBS- and total SOV-treated groups) or 2 weeks (for total SOVs from WT and total SOVs from miR-143/145 KO mice). Defect areas were measured using ImageJ. Treatment of miR-143/145-deleted SOVs in vitro Primary osteoblasts from WT and miR-143/145 Osx −/− female mice were cultured for 14 days. SOVs were collected and named WT-SOV and KO-SOV, respectively. Primary osteoblasts from WT female mice were cultured for 6 days and treated with PBS, WT-SOV or KO-SOV. RNA extraction was performed 2 days after treatment. Statistics and reproducibility Differences between two groups were analyzed using two-tailed paired, unpaired, or Welch’s t -tests. Differences among three or more groups were analyzed by one-way analysis of variance (ANOVA) with Dunnett’s multiple comparison post hoc test. 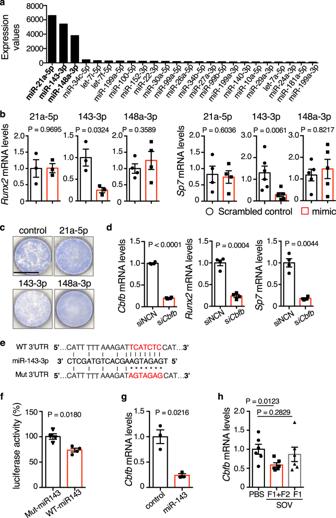Fig. 4: SOV-derived miR-143-3p inhibits osteoblast differentiation by targetingCbfbmRNA. aNext-generation sequencing-mediated miRNA profiling of SOVs. Top-ranked expression values of miRNAs in SOVs from primary osteoblasts of 10 Col2.3-ECFP mice.bRunx2andSp7mRNA levels in MC3T3-E1 cells transfected with scrambled, miR-21a-5p, miR-143-3p, or miR-148a-3p mimics (TheRunx2expression in miR-21a-5p and miR-143-3p groups:n= 3; theRunx2expression in a miR-148a-3p group and theSp7expression in a miR-21a-5p group:n= 4; theSp7expression in a miR-148a-3p group:n= 5; theSp7expression in a miR-143-3p group:n= 6 independent experiments, respectively).cRepresentative images of ALP activity in MC3T3-E1 cells transfected with scrambled, miR-21a-5p, miR-143-3p, or miR-148a-3p mimics. Scale bar: 10 mm.dCbfb,Runx2, andSp7mRNA levels in MC3T3-E1 cells transfected with siRNA negative control orCbfbsiRNA. siNCN: siRNA negative control; siCbfb:CbfbsiRNA (n= 4 independent experiments). The exactpvalue of theCbfbexpressioin: 2.34811−9.eCbfb3′ UTR constructs cloned into luciferase reporter vectors. WT 3′ UTR: wild-type sequence of theCbfb3′ UTR; miR-143-3p: miR-143-3p sequence; Mut 3′ UTR: mutant sequence of theCbfb3′ UTR.fPercentages of luciferase activity. Mut-miR143: mutatedCbfbconstruct with miR-143-3p mimics; WT-miR143: WTCbfbconstruct with miR-143-3p mimics (n= 4 independent experiments).gCbfbmRNA levels in MC3T3-E1 cells treated with scrambled control or miR-143-3p mimics. Control: scrambled controls; miR-143: miR-143-3p mimics (n= 3 independent experiments).hCbfbmRNA levels in primary osteoblasts treated with PBS, total SOVs (F1 + F2), or SOV-F1 (n= 6 biological replicates per group). Data are means ± SEMs. Statistical significance was determined by two-tailed pairedt-test in (b,d,f,g) and by one-way ANOVA with Dunnett’s multiple comparison post hoc test in (h). Welch’s ANOVA followed by Bonferroni’s multiple comparisons test was used when the data demonstrated unequal variance. Statistical analyses were performed using Prism ver. 6 (GraphPad Software) and JMP16. Numbers of samples and animals are indicated in the figure legends. All data are representative of those of at least three independent experiments unless otherwise indicated. Biological replicates comprised samples from different mice. 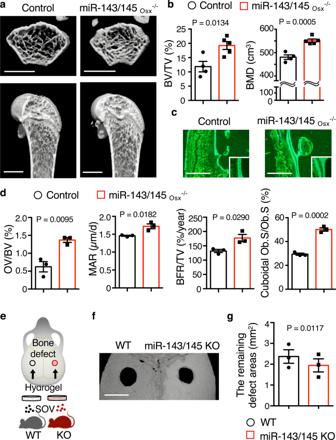Fig. 5: miR-143/145 conditional KO increases bone mass and promotes mineralization in mice. aRepresentative micro-CT images of the femurs of 9-week-old control (n= 4 biological replicates) and osteoblast-specific miR-143/145 KO (miR-143/145Osx−/−) mice (n= 5 biological replicates). Scale bars: 1000 μm.bMicro-CT-based assessment of metaphyseal regions of distal femurs of 9-week-old control (n= 4 biological replicates) and miR-143/145Osx−/−(n= 5 biological replicates) mice. BV: bone volume; TV: tissue volume; BMD: bone mineral density.c,dBone morphometric analysis of metaphyseal regions of distal femurs of 9-week-old control and miR-143/145Osx−/−mice (n= 3 biological replicates per group). Calcein double signals in a representative femur section from a control or miR-143/145Osx−/−mouse on cortical surfaces and magnified view (inset). Scale bars: 100 µm (c). Bone formation parameters (d). OV: osteoid volume; MAR: mineral apposition rate; BFR: bone formation rate; Ob.S: osteoblast surface.eTransplantation model of calvarial defects. Artificial bilateral defects on mouse calvaria were treated with total SOVs from miR-143/145 KO or WT mice.fRepresentative micro-CT image of calvarial defects at 2 weeks after treatment with SOVs from miR-143/145 KO or WT mice (n= 3 biological replicates per group). Scale bar: 2000 µm.gRemaining defect areas. miR-143/145 KO: mice treated with total SOVs from miR-143/145 KO mice; WT: mice treated with SOVs from WT mice (n= 3 biological replicates per group). Data are means ± SEMs. Statistical significance was determined by two-tailed unpairedt-test in (b,d) or by two-tailed pairedt-test in (g). 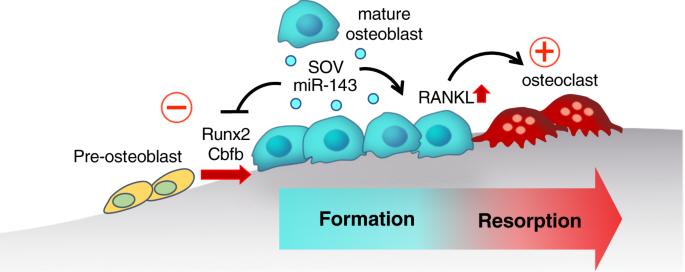Fig. 6: Graphical abstract of the role of small osteoblast vesicles in bone remodeling. Interactions among mOBs via SOVs inhibit osteoblastic bone formation and stimulate osteoclast formation, thus switching from the bone formation phase to the bone resorption phase. We estimated the required sample sizes by considering variations and means, and sought to reach reliable conclusions using sample sizes that were as small as possible. Reporting summary Further information on research design is available in the Nature Research Reporting Summary linked to this article.